Evolution of gene network activity by tuning the strength of negative-feedback regulation Despite the examples of protein evolution via mutations in coding sequences, we have very limited understanding on gene network evolution via changes in cis -regulatory elements. Using the galactose network as a model, here we show how the regulatory promoters of the network contribute to the evolved network activity between two yeast species. In Saccharomyces cerevisiae , we combinatorially replace all regulatory network promoters by their counterparts from Saccharomyces paradoxus , measure the resulting network inducibility profiles, and model the results. Lowering relative strength of GAL80 -mediated negative feedback by replacing GAL80 promoter is necessary and sufficient to have high network inducibility levels as in S. paradoxus . This is achieved by increasing OFF-to-ON phenotypic switching rates. Competitions performed among strains with or without the GAL80 promoter replacement show strong relationships between network inducibility and fitness. Our results support the hypothesis that gene network activity can evolve by optimizing the strength of negative-feedback regulation. Cells often use gene networks to respond to their environments [1] , [2] , [3] , [4] , [5] . During evolution, selective pressures act on gene network activity and networks with optimal activity levels can confer fitness advantages on their host organisms [6] . Uncovering the mechanisms of gene network evolution is of fundamental importance in biology; yet, we have little knowledge about how cells rewire their networks to better adapt to the environment [7] , [8] . This lack of understanding is compounded by the presence of feedback-mediated nonlinear interactions among the components of gene networks; such interactions make it challenging to analyse input–output relationships and to ultimately dissect the mechanisms of gene network evolution. To investigate whether there are key network components or motifs that could drive the evolution of gene network activity between different species, we used the galactose utilization pathway [4] , [9] as our model network and the yeast species S. cerevisiae and S. paradoxus as our model organisms. S. paradoxus is the closest relative of S. cerevisiae and the GAL network is an evolutionarily preserved network between the two species [6] , [10] . All four regulatory proteins (Gal2p, Gal3p, Gal4p and Gal80p) of the network have the same functional roles [10] in both species, and there are high levels of homology between the GAL network promoters and genes from both species. In the GAL network, the galactose signal propagates through a four-stage signalling cascade [4] , [9] , [11] , [12] . The galactose transporter Gal2p imports extracellular galactose into the cell, and intracellular galactose binds to and activates the signal transducer Gal3p. The activated Gal3p then binds to the inhibitor Gal80p. As a result, the transcriptional activator Gal4p is released from the inhibitory effect of Gal80p and activates expression of the network genes, including GAL2 , GAL3 , GAL80 and GAL1 . The activator Gal4p itself is constitutively expressed and it has a conserved binding motif on all GAL network promoters from both species [10] . Due to the presence of Gal4p binding sites on the network promoters from both species, the GAL network in both species displays the same network architecture built by two positive (through GAL2 and GAL3 ) and one negative (through GAL80 ) feedback loops. Here we study whether or not cross-species differences in the regulatory promoters of a natural gene network can be sufficient to explain the differences in the evolved activity of the network. Using the GAL network of yeast S. cerevisiae and S. paradoxus , and performing single-cell level experiments and analyses, we measure the contribution of each species-specific network promoter on the evolved activity of the GAL network. Among the four regulatory promoters of the network, the cross-species difference in the strength of the GAL80 promoter is the highest. Genetically swapping the GAL80 promoter is necessary and sufficient to alter the activity of the network between the two yeast species. This is achieved by changing the phenotypic switching rates between the OFF and ON state of the bimodal network. Strong connections between network activity and fitness are observed when competition experiments are performed among strains with or without the GAL80 promoter replacement. A quantitative model provides mechanistic insights into our experimental results. Cross-species comparison of GAL network activity To compare the activity of the GAL network ( Fig. 1a ) between the two yeast species, we used the yellow fluorescent protein (YFP) driven by the GAL1 promoter as our single-cell level reporter in wild-type haploid S. cerevisiae and S. paradoxus strains. Each strain contained its own endogenous GAL1 promoter to drive YFP. Then, we measured P GAL1 –YFP expression profiles at different galactose concentrations by using flow cytometry after 22 h of cell growth. The activity of the GAL network in both species displayed bimodal profiles. In these experiments, to provide similar growth rates ( Supplementary Fig. 1 ) for the OFF and ON cells, we used 0.1% mannose as an additional, non-inducing neutral sugar. For bimodal expression profiles [4] , [9] , [13] , [14] , [15] ( Fig. 1b ), the fraction of cells occupying the ON-state is defined as the inducibility of the network [9] . We used inducibility of the GAL network as the quantitative phenotypic trait to compare between the two yeast species. We observed distinctly different network inducibility profiles between the two wild-type strains ( Fig. 1c ). The activity of the GAL network in S. paradoxus could be turned ON at a much lower galactose concentration. 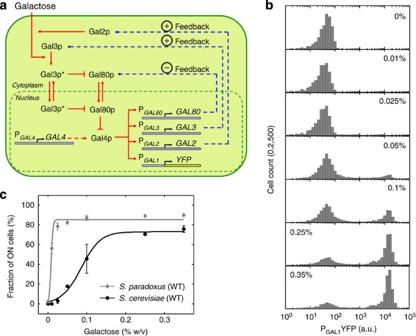Figure 1: Comparison of GAL network activity between two yeast species. (a) Network architecture built by the four regulatory genes. The red lines denote the four-stage signalling cascade. The galactose-bound state of Gal3p is denoted by Gal3p*. Pointed and blunt red arrows reflect activation and inhibition, respectively. The dashed blue arrows denote feedback loops established by Gal2p, Gal3p and Gal80p. The dashed red arrow represents the constitutive expression of the Gal4 proteins. The double red arrows denote translocation of Gal80p and Gal3p* between cytoplasm and nucleus. (b) Histograms showing the inducibility profile of the wild-typeS. cerevisaeGAL network at different galactose concentrations. a.u., arbitrary units. (c) Inducibility as a function of galactose concentration for wild-type GAL networks inS. cerevisaeandS. paradoxus. The solid lines (guides to the eye) are constructed by fitting a sigmoidal function to the data. Error bars indicate s.e.m. (N=2). Figure 1: Comparison of GAL network activity between two yeast species. ( a ) Network architecture built by the four regulatory genes. The red lines denote the four-stage signalling cascade. The galactose-bound state of Gal3p is denoted by Gal3p*. Pointed and blunt red arrows reflect activation and inhibition, respectively. The dashed blue arrows denote feedback loops established by Gal2p, Gal3p and Gal80p. The dashed red arrow represents the constitutive expression of the Gal4 proteins. The double red arrows denote translocation of Gal80p and Gal3p* between cytoplasm and nucleus. ( b ) Histograms showing the inducibility profile of the wild-type S. cerevisae GAL network at different galactose concentrations. a.u., arbitrary units. ( c ) Inducibility as a function of galactose concentration for wild-type GAL networks in S. cerevisae and S. paradoxus . The solid lines (guides to the eye) are constructed by fitting a sigmoidal function to the data. Error bars indicate s.e.m. ( N =2). Full size image Replacing the promoters of the S. cerevisiae GAL network To elucidate which network components or interaction topologies were responsible from the observed differences in network inducibility profiles, we combinatorially replaced each regulatory promoter of the GAL network in haploid S. cerevisiae by its homologous counterpart from S. paradoxus , obtaining 16 different haploid S. cerevisiae strains carrying one, two, three or all four GAL regulatory promoters replaced by their counterparts from S. paradoxus. We focused on the replacement of the regulatory promoters with the goal of finding out whether or not promoter replacements alone were sufficient to explain the cross-species differences in network inducibility profiles. The regulatory proteins from the two yeast species have high degrees of amino-acid sequence similarities (from 89.8 to 99.5%, Supplementary Methods ). However, this does not provide any evidence into their level of contribution to network evolution, since even single amino-acid substitutions can significantly change protein-binding rates. In making the promoter replacements, not to miss a potentially important regulatory site, we replaced the whole upstream intergenic regions. To preserve the potential genome location-specific effects and to prevent the introduction of foreign restriction sites, we made the promoter replacements in a ‘scar-free’ manner by using the URA -5FOA counter-selection method [16] (Methods). Replacing the promoters at their endogenous locations is essential for a faithful cross-species comparison of promoter strengths. We chose the haploid S. cerevisiae as the host strain so that we could take advantage of the relatively high recombination rates that are necessary for the efficiency of the counter-selection method we used. Using one-strain background as the host and replacing the promoters in a systematic way were important for controlled and accurate interpretations of the experimental results. Compared with the wild-type S. cerevisiae profile, replacing the GAL80 promoter caused a 44% increase in the inducibility profile (when averaged over seven induction conditions), whereas replacing the GAL3 promoter decreased the inducibility by 17% ( Fig. 2a , columns 1–2). Replacing the GAL2 or GAL4 promoter did not have a significant effect on network inducibility (1 and 2% average changes were observed for GAL2 and GAL4 , respectively). Since GAL80 ( GAL3 ) is a negative (positive) regulator in the GAL network, these results showed us that the S. paradoxus GAL80 and GAL3 promoters were weaker in strength compared with their counterparts from S. cerevisiae . We interpreted these experimental results by building an effective quantitative model ( Supplementary Methods , Supplementary Tables 1–4 ). By following a mean-field theoretical approach to predict the fraction of ON cells and by using only one-fit parameter representing the strength of each replaced promoter, we performed a least-squares fit between our model and five inducibility profiles shown in Fig. 2a (columns 1–2). To test the predictive power of our model, we used it to predict the remaining 11 experimental inducibility profiles in Fig. 2a (columns 3–5) without using any free parameters. We saw a high degree of agreement between the experimental results and model predictions. 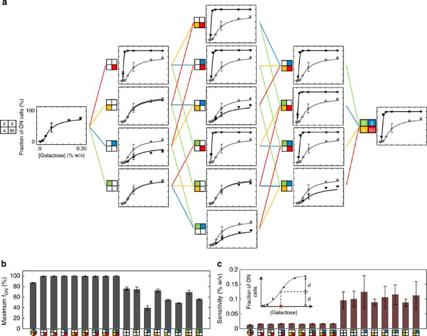Figure 2: Combinatorial promoter replacements inS. cerevisaeand their effect on network inducibility and sensitivity. (a) The inducibility profiles of the promoter-replaced GAL network (black) relative to the wild-type profile (black on the leftmost panel, grey on the rest). The thick solid lines reflect the predictions of the model based on the best fit to the data. The genetic background of each haploidS. cerevisaestrain is specified by a big square at its immediate left. The small squares represent the four regulatory promoters replaced (if coloured) by theirS. paradoxuscounterparts. A line between two strains indicates that the two genetic backgrounds differ by only one promoter replacement and the colour of the line codifies the replaced promoter (blue for PGAL3, red for PGAL80, green for PGAL2, yellow for PGAL4). Error bars indicate s.e.m. (N=2). (b) Maximal inducibility levels (fraction of ON cells at 0.35% galactose) across all genetic backgrounds. Error bars indicate s.e.m. (N=2). The maximum inducibility of the wild-typeS. paradoxusGAL network is shown at far left (coloured circle) for comparison purposes. (c) Sensitivity to galactose induction across all genetic backgrounds. Error bars indicate s.e.m. (N=2). The inset shows how sensitivity is quantified: the concentration of galactose necessary for half-maximal inducibility (the solid line represents the fit result). The sensitivity of the wild-typeS. paradoxusGAL network is shown at far left (coloured circle). The PGAL80replacement (red square) is necessary and sufficient for obtaining similar inducibility and galactose sensitivity profiles between the two yeast species. Figure 2: Combinatorial promoter replacements in S. cerevisae and their effect on network inducibility and sensitivity. ( a ) The inducibility profiles of the promoter-replaced GAL network (black) relative to the wild-type profile (black on the leftmost panel, grey on the rest). The thick solid lines reflect the predictions of the model based on the best fit to the data. The genetic background of each haploid S. cerevisae strain is specified by a big square at its immediate left. The small squares represent the four regulatory promoters replaced (if coloured) by their S. paradoxus counterparts. A line between two strains indicates that the two genetic backgrounds differ by only one promoter replacement and the colour of the line codifies the replaced promoter (blue for P GAL3 , red for P GAL80 , green for P GAL2 , yellow for P GAL4 ). Error bars indicate s.e.m. ( N =2). ( b ) Maximal inducibility levels (fraction of ON cells at 0.35% galactose) across all genetic backgrounds. Error bars indicate s.e.m. ( N =2). The maximum inducibility of the wild-type S. paradoxus GAL network is shown at far left (coloured circle) for comparison purposes. ( c ) Sensitivity to galactose induction across all genetic backgrounds. Error bars indicate s.e.m. ( N =2). The inset shows how sensitivity is quantified: the concentration of galactose necessary for half-maximal inducibility (the solid line represents the fit result). The sensitivity of the wild-type S. paradoxus GAL network is shown at far left (coloured circle). The P GAL80 replacement (red square) is necessary and sufficient for obtaining similar inducibility and galactose sensitivity profiles between the two yeast species. Full size image To comprehensively explore the effect of all possible promoter replacements on the activity of the GAL network, we measured the inducibility profiles of all 16 strains ( Supplementary Table 5 ), ordered the measurements in 4 combinatorial groups indicating the number of replaced promoters in a single strain, and compared the profiles with one another. Figure 2a–c depicts the importance of GAL80 promoter in affecting the inducibility profiles and galactose sensitivity levels across all 16 strains. 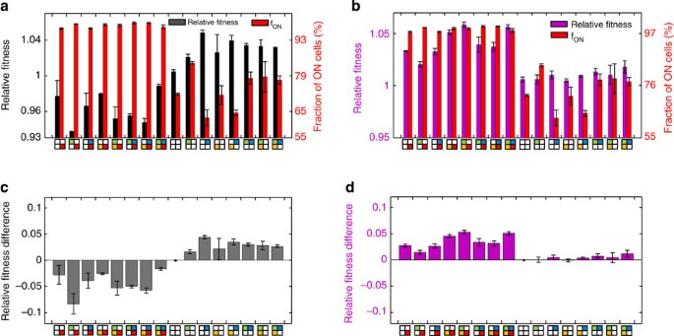Figure 5: The effect of promoter replacements on cellular fitness profiles. (a) Relative fitness of each YFP-containingS. cerevisiaestrain relative to a wild-typeS. cerevisiaestrain carrying the constitutively expressed tdTomato reporter. Strains competed for 48 h in minimal media containing 0.01% galactose and 0.03% mannose as carbon sources. The dark grey bars indicate the relative fitness level of each strain. The red bars represent the fraction of ON cells (of the YFP-containing strains) measured at 48 h. At the beginning of the competition, the fraction of ON cells was 0%. (b) Relative fitness values of the strains in minimal media environment containing 1% galactose as the sole carbon source. Competing strains of the first environment (a) were transferred to this second environment and competitions lasted for another 44 h. The fractions of ON cells (of the YFP-containing strains) at the beginning of this environmental exposure are plotted using red colour and the purple colour represents the relative fitness levels. All YFP-expressing strains were measured to have 100% ON cells at the end of the 44 h duration. (c,d) For the first (c) and second (d) environment, the relative fitness differences between each YFP-containing strain and the wild-type strain containing YFP. In all panels (a–d), error bars indicate s.e.m. (N=2). In all panels (a–d), the genetic background of each haploidS. cerevisaestrain is specified by the squares below the panels. The small squares represent the four regulatory promoters replaced (if coloured) by theirS. paradoxuscounterparts. The colour coding is: blue for PGAL3, red for PGAL80, green for PGAL2, yellow for PGAL4. The galactose sensitivity levels were measured by quantifying the galactose concentration corresponding to half-maximal network induction for each strain ( Fig. 2c , inset). Even though replacing the GAL3 promoter alone had a negative effect on network inducibility, whenever we replaced both GAL80 and GAL3 promoters in a single strain, the effect of GAL80 was dominant over the effect of GAL3 in terms of affecting the inducibility profiles or galactose sensitivity levels. Replacing GAL2 or GAL4 did not change these profiles in a significant manner across different strains. Figure 2b,c also shows the results from the wild-type S. paradoxus GAL network (coloured circle at left). We found that replacing only the GAL80 promoter was necessary and sufficient to move the inducibility and galactose sensitivity levels between the two wild-type profiles from the two species. Relative contribution of the promoters to network activity To quantify the relative significance of each replaced promoter in changing the wild-type inducibility levels of the S. cerevisiae GAL network, we used a metric ( Supplementary Methods ) and quantified the average contribution of each promoter replacement to inducibility and galactose sensitivity across all relevant strains. For the phenotype of inducibility, the metric calculated the differences between the inducibility levels of genetically neighbouring strains and averaged the results ( Fig. 3a ). The effect of the GAL80 promoter on inducibility was the largest (49.73%), compared with the effects of GAL2 (0.46%), GAL3 (−6.37%) or GAL4 (0.76%). For the phenotype of galactose sensitivity, the metric quantified the differences between the galactose sensitivity levels of genetically neighbouring strains and averaged the results ( Fig. 3b ). The effect of the GAL80 promoter on galactose sensitivity was the largest (−0.0111%), compared with the effects of GAL2 (0.0004%), GAL3 (0.0021%) or GAL4 (−0.0002%). 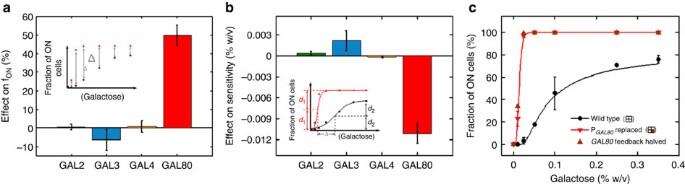The results from these analyses reaffirmed the importance of the GAL80 promoter over the other network promoters in terms of affecting the phenotypes. Figure 3: Average contribution of promoter replacements to network inducibility and galactose sensitivity. (a) Average contributions to network inducibility. Separately for each promoter, all genetic backgrounds in which that promoter was replaced were identified, corresponding to 8 out of 16 strain backgrounds. Inducibility values of the strains that carry theS. cerevisaeversion of a specific promoter were subtracted (as the inset shows) from the inducibility values of the strains carrying theS. paradoxusversion of that promoter in an otherwise identical genetic background and these differences were averaged for each promoter. Error bars indicate s.e.m. (N=2) of this averaging. (b) Average contributions to galactose sensitivity. Differences in galactose sensitivity were measured and averaged among different genetic backgrounds as described in (a). Error bars indicate s.e.m. (N=2). Inset show how the sensitivity difference between the fitted inducibility profiles of two strains would be obtained. The PGAL80replacement causes the largest change in inducibility and galactose sensitivity. (c) Inducibility profiles of the wild type, PGAL80replaced andGAL80feedback-halved GAL networks inS. cerevisae. Error bars indicate s.e.m. (N=2). Solid lines indicate model results. TheGAL80feedback-halved profile was obtained from a diploid strain carrying one copy of theGAL80gene in an otherwise wild-type background by using the same PGAL1-YFP reporter. Figure 3: Average contribution of promoter replacements to network inducibility and galactose sensitivity. ( a ) Average contributions to network inducibility. Separately for each promoter, all genetic backgrounds in which that promoter was replaced were identified, corresponding to 8 out of 16 strain backgrounds. Inducibility values of the strains that carry the S. cerevisae version of a specific promoter were subtracted (as the inset shows) from the inducibility values of the strains carrying the S. paradoxus version of that promoter in an otherwise identical genetic background and these differences were averaged for each promoter. Error bars indicate s.e.m. ( N =2) of this averaging. ( b ) Average contributions to galactose sensitivity. Differences in galactose sensitivity were measured and averaged among different genetic backgrounds as described in (a). Error bars indicate s.e.m. ( N =2). Inset show how the sensitivity difference between the fitted inducibility profiles of two strains would be obtained. The P GAL80 replacement causes the largest change in inducibility and galactose sensitivity. ( c ) Inducibility profiles of the wild type, P GAL80 replaced and GAL80 feedback-halved GAL networks in S. cerevisae . Error bars indicate s.e.m. ( N =2). Solid lines indicate model results. The GAL80 feedback-halved profile was obtained from a diploid strain carrying one copy of the GAL80 gene in an otherwise wild-type background by using the same P GAL1 -YFP reporter. Full size image S. paradoxus P GAL80 is weaker than S. cerevisiae P GAL80 Since GAL80 promoter is part of the main negative-feedback loop in the GAL network ( Fig. 1a ), the high inducibility levels observed when this promoter was replaced suggested that the S. paradoxus GAL80 promoter was weaker than its S. cerevisiae counterpart, and this expectation was verified by our model. However, the high inducibility levels could also result from foreign cis -regulatory elements specific to S. paradoxus . To experimentally prove that the weaker promoter strength of the S. paradoxus GAL80 promoter is the cause of the high inducibility levels, we halved the strength of the S. cerevisiae GAL80 promoter in a diploid S. cerevisiae strain (by deleting one of the two GAL80 genes) and experimentally measured its inducibility profile ( Fig. 3c ). The resulting profile was very similar to the profile obtained from the strain carrying the S. paradoxus GAL80 promoter. Regarding having a diploid background for this experiment, previous work [9] showed that the activity of the S. cerevisiae GAL network was similar in haploid and diploid backgrounds. In addition, we performed quantitative PCR experiments on two haploid S. cerevisiae strains, one strain carrying the endogenous GAL80 promoter and the other one carrying its S. paradoxus counterpart. We saw that the S. paradoxus GAL80 promoter was 32% weaker than its S. cerevisiae counterpart ( Supplementary Table 6 ). To further explore the effect of the negative-feedback strength modulation on the network inducibility, we used our model without any extra fit parameters and changed the negative-feedback strength from wild-type level to 20% of the wild type ( Supplementary Fig. 2 ). The lower the feedback strength was, the sharper the inducibility profiles turned out to be, as expected. To find out which part of the S. paradoxus GAL80 promoter makes it weaker in strength compared with its S. cerevisiae counterpart, we constructed synthetic ‘hybrid’ promoters by using parts from the two endogenous versions of the GAL80 promoter. Then, in the wild-type S. cerevisiae strain, we replaced its endogenous GAL80 promoter with these hybrid promoters and measured the resulting network inducibility profiles ( Supplementary Fig. 3 , brown data points). All hybrid promoters still contained the single binding site for the binding of the Gal4 proteins on them. The first hybrid promoter had base pairs (1–139) from S. paradoxus and (140–282) from S. cerevisiae , giving rise to a network inducibility profile similar to the one observed in wild-type S. cerevisiae ( Supplementary Fig. 3 , black data points). Having the second half (141–288 bp) of the hybrid promoter from S. paradoxus , and the first half (1–140 bp) from S. cerevisiae , reverted the phenotype to the one observed from the endogenous S. paradoxus GAL80 promoter, indicating that the cross-species strength difference is caused by differences in the second half of the GAL80 promoter. Further analysis on the other hybrid promoters showed us that the final ~100 bp region (181–288 bp, hybrid 4) of the GAL80 promoter was essential to dictate the network inducibility profile. Further reducing the length of this region made the profile become less similar to the one obtained from the endogenous S. paradoxus GAL80 promoter. Inspecting the final 100 bp region of the promoter, we picked two ‘point mutations’, one corresponding to the introduction of a 4 bp region (TTCC) and the other being an A-to-G transition. To see if these mutations could revert the phenotype on their own, we constructed two more strains (WP0101, WP0103) and measured the resulting inducibility profiles ( Supplementary Fig. 3 , bottom two panels). The effect of these mutations was not strong enough to revert the inducibility profile. Our results show that the cross-species strength difference between the two endogenous GAL80 promoters was due to multiple mutations (seven transition mutations, as well as a 4 bp insertion) localized in the final ~100 bp region of the promoter. Since the size of the hybrid promoters are similar, as well as the distance between the Gal4 binding site and the end of the promoters, our results indicate that these mutations between the two endogenous promoters likely affect the efficiency of the transcriptional initiation and/or elongation processes, perhaps by altering the looping dynamics of the promoter. Expressing S. paradoxus Gal4 proteins in S. cerevisiae As another important control, we also considered the possibility that Gal4 proteins from the two yeast species could interact differently with the network promoters and this might affect the network indicibility levels. To test this possibility, we replaced the GAL4 gene of S. cerevisiae by its counterpart from S. paradoxus . We made this genetic replacement in both the wild-type S. cerevisiae background and the S. cerevisiae background having all four regulatory promoters replaced by their S. paradoxus counterparts. We saw no significant differences between the experimental inducibility profiles of the strains carrying either the S. cerevisiae or S. paradoxus Gal4 proteins ( Supplementary Fig. 4 ). Relative amounts of the network proteins in the two species To have a direct experimental understanding on the relative concentrations of the network proteins between the two wild-type yeast species, we performed western blot experiments ( Supplementary Fig. 5 ). When the network was induced with galactose, all four regulatory proteins of the network showed lower expression levels in S. paradoxus compared to the levels in S. cerevisiae . The relative cross-species reduction in protein production rates ( θ ) were 2.8-fold for Gal2, 2-fold for Gal3 and 1.3-fold for Gal4. For the Gal80 proteins, the cross-species reduction in the production rate was the highest at 6.5-fold. On the basis of fitting our model to the inducibility data obtained from the promoter-swapped S. cerevisiae strains ( Fig. 2a ), the relative reduction in cross-species protein production rates our model predicted were 1.38-fold for Gal2, 1.33-fold for Gal3, 0.92-fold for Gal4 and 2.45-fold for Gal80 ( Supplementary Table 3 ). The experimentally obtained and model-predicted numbers agree on three fronts. First, Gal80 protein expression rates are the most different between the two species. Second, Gal4 production rates are the most similar and the lowest compared with the other network proteins. Third, the production rates of the three network-regulated proteins (Gal2, Gal3 and Gal80) are smaller for S. paradoxus compared with S. cerevisiae . Previous work [9] has shown that the activity of the S. cerevisiae GAL network was compensated or invariant to coordinated changes in the production rates of network proteins. For example, in a diploid strain background, reducing the number of copies of all regulatory network genes from two copies to one copy does not alter the inducibility profile of the network. The same work also showed that GAL80 and GAL3 genes made the most important contributions to this compensated phenotype due to the way they are wired to the network architecture (which is the same in S. cerevisiae and S. paradoxus ). Therefore, in evaluating the abundance of network proteins in the two yeast species, one has to keep in mind that the relative abundance of the proteins, as opposed to absolute numbers, is essential in affecting the network inducibility levels in each species. To show this effect quantitatively, we ran simulations by varying the absolute and relative protein production rates for the two key network proteins, Gal80 and Gal3. As shown in Supplementary Fig. 6 , as long as the protein production rates for Gal80 and Gal3 are similar, the network displays similar inducibility profiles irrespective of the differences in the absolute values of the production rates. However, when the two proteins are produced at different rates, the relative difference has a big effect on the network inducibility profile. Next, under the guidance of this understanding, we evaluated the model using the experimentally obtained protein production rates in S. paradoxus . Without using any fit parameters, we fed these values into our model and plotted the network inducibility profile ( Supplementary Fig. 7 , red dotted line). The resulting profile turned out to be easily inducible, similarly to the experimental profile ( Supplementary Fig. 7 , grey symbols). To show that it is the relative difference between the Gal80 and Gal3 production rates (232 versus 749 proteins per hour) that causes this easily inducible phenotype, we generated another inducibility profile with the two production rates equal to each other at 749 proteins per hour (green dotted line). As expected, this profile was much less inducible (44.5% less than the red dotted profile, when averaged over seven galactose induction levels) and it was more similar to the S. cerevisiae profile (black symbols). Cloning the S. cerevisiae GAL80 promoter into S. paradoxus To see how the S. paradoxus GAL network activity would change due to a promoter swap at the GAL80 promoter locus, we replaced the endogenous GAL80 promoter in S. paradoxus by the S. cerevisiae GAL80 promoter. As Supplementary Fig. 8a,b show, the resulting network inducibility profile (green) was 54% lower compared with the profile displayed by the wild-type S. paradoxus (grey), indicating the stronger nature of the S. cerevisiae GAL80 promoter. A similar level of change (44%, Supplementary Fig. 8b , red) had been observed when we measured the average inducibility difference between two S. cerevisiae strains carrying the two versions of the GAL80 promoter, indicating that the S. cerevisiae GAL80 promoter is stronger compared with its counterpart and the effect of this strength difference on network inducibility is species independent. To prove that the S. paradoxus cells carrying the S. cerevisiae GAL80 promoter indeed have more Gal80 proteins compared with the wild-type S. paradoxus cells, we performed western blot experiments on the two S. paradoxus strains carrying one of the two versions of the GAL80 promoter ( Supplementary Fig. 8c,d ). Between the two strains, we observed an approximately fourfold average difference in the Gal80 protein levels of the ON cells, verifying that the S. cerevisiae GAL80 promoter was indeed stronger than its S. paradoxus counterpart. Effect of promoter replacements on phenotypic switching rate Next we explored how the experimentally measured expression distributions (for example, Fig. 1b , for the wild-type strain) are shaped by the phenotypic switching rates between the OFF and ON states of the GAL network [4] , [17] . An efficient experimental way to quantify switching rates is to subject the network to different initial overnight growth conditions, separately induce the resulting network profiles for a fixed duration, measure the resulting expression histograms and use mathematical analysis to extract the switching rates ( Supplementary Methods ). For each galactose induction level used, Fig. 4 shows the values of the phenotypic switching rates between the OFF and ON states of the network. All GAL80 promoter-replaced strains displayed relatively high OFF-to-ON switching rates. In the 0% galactose environment, relatively high ON-to-OFF switching rates (with low OFF-to-ON rates) are a reflection of all cells being in the OFF state of the network after 22 h of growth. To find out if lowering the strength of the S. cerevisiae GAL80 negative-feedback loop could explain the high OFF-to-ON switching rates displayed by the GAL80 promoter-replaced strains, we measured the switching rates of the strain which was halved in the strength of its GAL80 negative feedback. The 50% reduction in the negative-feedback strength was indeed able to show us higher OFF-to-ON switching rates ( Supplementary Fig. 9 ). To see how the synthetic hybrid promoters we constructed affect the switching rates of their host strains, we included them in our switching rates analysis. As Supplementary Fig. 10 shows, the hybrid promoter carrying the last ~100 bp of the S. paradoxus GAL80 promoter (third from left in the figure) gave rise to a switching rates profile that was similar to the profile caused by the endogenous S. paradoxus GAL80 promoter (first from left). Supplementary Fig. 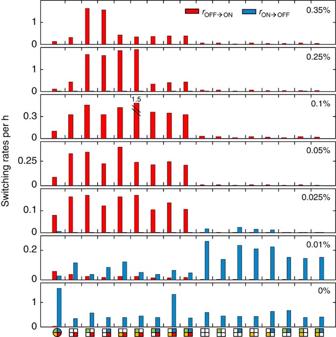11 shows how we tested the method used in measuring the switching rates. Figure 4: The effect of promoter replacements on the rates of phenotypic switching between the two expression states of the GAL network. At each indicated galactose concentration, OFF-to-ON state (red) and ON-to-OFF state (blue) switching rates were measured for each strain. One of the bars was plotted discontinuously and the actual switching rate (1.5) for that strain/condition is shown on the bar. The genetic background of each haploidS. cerevisaestrain is specified by the squares below the data panels. The small squares represent the four regulatory promoters replaced (if coloured) by theirS. paradoxuscounterparts. The colour coding is: blue for PGAL3, red for PGAL80, green for PGAL2, yellow for PGAL4. The coloured circle at far left represents the wild-typeS. paradoxusGAL network. Figure 4: The effect of promoter replacements on the rates of phenotypic switching between the two expression states of the GAL network. At each indicated galactose concentration, OFF-to-ON state (red) and ON-to-OFF state (blue) switching rates were measured for each strain. One of the bars was plotted discontinuously and the actual switching rate (1.5) for that strain/condition is shown on the bar. The genetic background of each haploid S. cerevisae strain is specified by the squares below the data panels. The small squares represent the four regulatory promoters replaced (if coloured) by their S. paradoxus counterparts. The colour coding is: blue for P GAL3 , red for P GAL80 , green for P GAL2 , yellow for P GAL4 . The coloured circle at far left represents the wild-type S. paradoxus GAL network. Full size image Fitness differences among promoter-replaced strains To understand how differences in network inducibility levels translate into fitness differences across different strains, we performed competition experiments (Methods). In two different growth environments containing low or high galactose, we measured the fitness of each of the 16 strains (containing YFP) relative to a wild-type S. cerevisiae strain carrying a constitutively expressed tdTomato reporter ( Supplementary Fig. 12 ). The first environment contained 0.01% galactose and 0.03% mannose as the carbon sources, while the second one contained 1% galactose. We supplemented the first environment with low mannose as 0.01% galactose was too low to support cell growth. Since the first environment was low in galactose, we hypothesized that a strain having relatively more cells in the ON state of the GAL network would suffer from a fitness cost due to the burden of gene expression when there is not much galactose to metabolize. In the high-galactose environment, on the other hand, we expected a positive relationship between having higher fraction of ON cells and displaying higher fitness values, as high galactose levels would be beneficial for the ON cells. To test these hypotheses, we ran 16 separate competition experiments in duplicate for 48 h in the first environment. Then, we changed the environment to the second type and continued these competitions for another 44 h. We took FACS snapshots to quantify YFP versus tdTomato fractions at the beginning and at the end of each environmental exposure, measured cell densities and diluted the cultures as necessary to keep the densities low, and entered these FACS and OD 600 measurements into a metric [18] to quantify relative fitness values across the 16 genetic backgrounds (Methods). Figure 5 and Supplementary Fig. 13 show the results from these fitness measurements. In the first environment, all GAL80 promoter replaced strains suffered from a fitness cost relatively to the wild-type strain ( Fig. 5a dark grey, and Fig. 5c ). As hypothesized, we saw a reverse relationship between the fitness levels and the fraction of ON cells ( Fig. 5a , red) measured at the end of the first environment ( t =48 h). The fractions of ON cells at t =0 were 0% due to the overnight growth in non-inducing mannose. In the second environment, the GAL80 promoter replaced strains displayed much higher fitness levels relative to the wild-type strain ( Fig. 5b purple and Fig. 5d ). As expected, we saw a positive relationship between the fitness levels and the fraction of ON cells ( Fig. 5b , red) measured at the beginning of the second environment. The ON fractions measured at the end of the second environment were all 100% due to the presence of 1% galactose as the sole carbon source, therefore the fitness differences observed in the second environment were due to the differences in the fraction of ON cells displayed at the beginning of the second environment. Figure 5: The effect of promoter replacements on cellular fitness profiles. ( a ) Relative fitness of each YFP-containing S. cerevisiae strain relative to a wild-type S. cerevisiae strain carrying the constitutively expressed tdTomato reporter. Strains competed for 48 h in minimal media containing 0.01% galactose and 0.03% mannose as carbon sources. The dark grey bars indicate the relative fitness level of each strain. The red bars represent the fraction of ON cells (of the YFP-containing strains) measured at 48 h. At the beginning of the competition, the fraction of ON cells was 0%. ( b ) Relative fitness values of the strains in minimal media environment containing 1% galactose as the sole carbon source. Competing strains of the first environment ( a ) were transferred to this second environment and competitions lasted for another 44 h. The fractions of ON cells (of the YFP-containing strains) at the beginning of this environmental exposure are plotted using red colour and the purple colour represents the relative fitness levels. All YFP-expressing strains were measured to have 100% ON cells at the end of the 44 h duration. ( c , d ) For the first ( c ) and second ( d ) environment, the relative fitness differences between each YFP-containing strain and the wild-type strain containing YFP. In all panels ( a – d ), error bars indicate s.e.m. ( N =2). In all panels ( a – d ), the genetic background of each haploid S. cerevisae strain is specified by the squares below the panels. The small squares represent the four regulatory promoters replaced (if coloured) by their S. paradoxus counterparts. The colour coding is: blue for P GAL3 , red for P GAL80 , green for P GAL2 , yellow for P GAL4 . Full size image These results provide quantitative understandings for the role of negative-feedback regulation in the evolved activity of a gene network across different species. Utilizing single-cell gene expression measurement techniques and quantitative modelling approaches, we uncovered that modulating the relative strength of the GAL80 negative-feedback loop was sufficient to make the inducibility profile of the GAL network be similar between the two yeast species S. cerevisiae and S. paradoxus . Measuring phenotypic switching rates between the OFF and ON expression states of the network further showed that the cross-species differences in network inducibility levels were due to the P GAL80 -caused differences in the OFF-to-ON switching rates. Finally, by performing competition experiments among strains that are different in terms of their GAL80 negative-feedback strength, we elucidated how feedback-strength differences could be translated into differences in fitness levels across the strains. Since several decades ago, mutations causing changes in gene expression regulation have been thought [19] , [20] , [21] to play important roles in evolutionary change, however, empirical evidence supporting such hypotheses has been emerging only recently [22] , [23] , [24] . Further, despite our increasing level of knowledge about the effect of feedback regulation [4] , [9] , [25] , [26] on gene network activity in single species and the effect of carbon metabolism gene regulation on fitness [27] , a systematic experimental and quantitative study characterizing the role of feedback-mediating promoters on the evolved activity of modular gene networks has been missing. At the cross section [28] of evolutionary biology and systems biology, our work provides an example to how gene network evolution could occur through tuning the strength of negative-feedback regulation. Construction of plasmids and yeast strains All S. cerevisiae strains used in this study were built on the MA0048 background. Complete descriptions of all strains can be found in Supplementary Table 5 . MA0048 is a haploid wild-type W303-background strain carrying the P GAL1 -YFP reporter construct in its ade2 locus. For this, KpnI −P GAL1 − BamHI and BamHI −YFP− EcoRI fragments were cloned into pRS402 plasmid backbone upstream of the CYC1 transcriptional terminator. The P GAL1 promoter sequence corresponds to the 669 bp region directly upstream of the start codon of the S. cerevisiae GAL1 gene. To construct the promoter-replaced haploid S. cerevisiae strains, the URA3 -5FOA counter-selection method was utilized [16] . The C. albicans URA3 cassette was PCR amplified from the pAG60 plasmid (Euroscarf) by using 5′ and 3′ primers carrying 60-bp homology to the region immediately up- and downstream of the replaced intergenic region. The transformed colonies were selected on plates missing uracil. As the second step of the construction process, each intergenic region was PCR-amplified from wild-type S. paradoxus by using 5′ and 3′ primers carrying 200-bp homology to the region immediately up- and downstream of the S. cerevisiae intergenic region carrying the C. albicans URA3 cassette. The transformed colonies were selected on plates containing 0.1% 5-FOA. The replacements were verified by PCR and sequenced to make sure that no mutations were introduced. The strains carrying the hybrid GAL80 promoters were constructed as described above, except that two strains (WP0089 and WP0090) were constructed by using the CRISPR/Cas9 gene editing approach [29] . For this, we integrated the Cas9 gene into our strain by using TRP1 as the marker. Following the introduction of a guide-RNA-targeted cut site in the GAL80 promoter, a double stranded PCR product carrying the intended hybrid promoter design was transformed into our strain and gave us the desired changes in the GAL80 promoter. Transformants carrying the correct change were verified by sequencing. For the strains carrying the replaced GAL4 gene, the URA3 cassette was integrated to replace the S. cerevisiae GAL4 gene by using 60-bp homology regions immediately before and after the GAL4 gene. The second step of the process included the transformation of the S. paradoxus GAL4 gene which was PCR-amplified by using 5′ and 3′ primers having 200-bp homology to the region immediately before and after the URA3 cassette. The transformed colonies were selected on plates containing 0.1% 5-FOA. The replacements were verified by PCR and sequenced to make sure that no mutations were introduced. To construct the wild-type S. paradoxus strain (MA0653) carrying the P GAL1 -YFP reporter (which uses S. paradoxus GAL1 promoter), KpnI −P GAL1 − BamHI and BamHI −YFP− EcoRI fragments were cloned into pRS402 plasmid backbone upstream of the CYC1 transcriptional terminator. The resulting plasmid was integrated into the P GAL1 locus of the wild-type S. paradoxus strain by using a previously described [30] transformation technique. The complete sequences of the GAL network promoters and genes from both yeast species are shown in Supplementary Methods . Growth conditions and media Cultures were grown in synthetic dropout media with the appropriate amino-acid supplements. During the overnight growth period (22 h in 30 °C shaker), 0.1% mannose was used as a non-inducing carbon source. For switching-rate measurement experiments, the overnight growth media contained either (0.1% mannose) or (0.1% mannose and 0.35% galactose) as carbon sources, so that we would obtain different initial conditions at the end of the overnight period ( Supplementary Methods ). The overnight growth period was followed by the induction period (22 h in 30 °C shaker), with cultures containing 0.1% mannose and 0–0.35% galactose as carbon sources. Mannose (0.1%) was used as a background carbon source ensuring similar growth rates across different galactose concentrations ( Supplementary Fig. 1 ). After the induction period, the expression distributions of ~10,000 cells were measured by flow cytometry (FACS-Verse; Becton Dickinson). Measurement results were quantitatively modelled ( Supplementary Methods , Supplementary Fig. 14 ). The OD 600 values at the end of the overnight and induction periods were kept low (OD 600 ~0.1) to prevent nutrient depletion. The culture volume was 10 ml during both overnight growth and induction periods. Growth conditions and procedures for competition experiments Throughout the competition experiments, cultures were grown in minimal media and the amino-acid content in the media was provided by the CSM-Ade mixture (complete supplement mixture minus adenine) supplemented with 0.01% adenine. Cultures were grown in a shaker set to 30 °C. Each of the 17 strains (16 strains with YFP and 1 with tdTomato) was separately grown overnight (22 h) in 10 ml minimal media containing 0.03% mannose as the carbon source. At the end of the overnight growth, the OD 600 density of the cells was ~0.1. Then, cells from each YFP-containing strain was separately mixed with cells from the tdTomato-containing strain by targeting 50–50% representation in the mixture. To obtain the relative fractions of the two cell types exactly, the cultures were analysed by the flow cytometer right after the mixing process. Following the mixing, the mixtures were diluted so that the OD 600 values after ~24 h would not exceed ~0.1. After ~24 h, the cultures were diluted once again in the same manner. Forty-eight hours after the initial mixing, another FACS measurement was taken to quantify the relative fraction of the two cell types. The OD 600 values at the time of this measurement were below 0.2. The media during the first 48 h (referred to as the first environment, Fig. 5a,c ) contained 0.01% galactose and 0.03% mannose, and the volume of the mixtures grown in the shaker was 5 ml. After the first environment, cells were transferred to the second environment ( Fig. 5b,d ) that contained 1% galactose as the sole carbon source. Cells were competed in this environment for another 44 h and relative fractions of the two cell types were quantified at the end of the competition. The OD 600 values during the growth in the second environment did not exceed 0.3 by diluting the cultures. The volume of the mixtures was 5 ml. For the YFP-expressing cells, the fraction of ON cells at the beginning of the first environment was 0% due to the overnight growth in non-inducing mannose. At the end of the second environment, the ON cell fractions were 100% for all YFP-containing strains, due to the presence of 1% galactose as the sole carbon source in the second environment. However, at the end of the first environment (or at the beginning of the second environment), the ON fractions were different between different strains ( Fig. 5a,b , red bars). For each environment, we quantified the relative fitness of each YFP-containing strain relative to the wild-type strain containing tdTomato. For this, we used the following metric [18] : where f i and f f are the fraction of YFP-containing cells at the beginning and at the end of each environment, while OD i and OD f are the initial and final densities of the mixture (by taking into account the dilutions). Fig. 5 and Supplementary Fig. 13 show the results from these analyses. How to cite this article: Peng, W. et al . Evolution of gene network activity by tuning the strength of negative-feedback regulation. Nat. Commun. 6:6226 doi: 10.1038/ncomms7226 (2015).